Maximizing the catalytic function of hydrogen spillover in platinum-encapsulated aluminosilicates with controlled nanostructures Hydrogen spillover has been studied for several decades, but its nature, catalytic functions and even its existence remain topics of vigorous debate. This is a consequence of the lack of model catalysts that can provide direct evidences of the existence of hydrogen spillover and simplify the catalytic interpretation. Here we use platinum encapsulated in a dense aluminosilicate matrix with controlled diffusional properties and surface hydroxyl concentrations to elucidate the catalytic functions of hydrogen spillover. The catalytic investigation and theoretical modelling show that surface hydroxyls, presumably Brønsted acids, are crucial for utilizing the catalytic functions of hydrogen spillover on the aluminosilicate surface. The catalysts with optimized nanostructure show remarkable activities in hydro-/dehydrogenation, but virtually no activity for hydrogenolysis. This distinct chemoselectivity may be beneficial in industrially important hydroconversions such as propane dehydrogenation to propylene because the undesired hydrogenolysis pathway producing light hydrocarbons of low value (methane and ethane) is greatly suppressed. Hydrogen spillover is the surface migration of activated H atoms from a hydrogen-rich metal cluster to the surface of a catalyst support where hydrogen dissociation is improbable. Since the discovery in the early 1960s [1] , [2] , hydrogen spillover has attracted the attention of many scientists, who have tried not only to explain it but also to exploit it for designing advanced catalysts with enhanced catalytic activity and lifetime [3] , [4] , [5] . Historically researchers have agreed on the existence of hydrogen spillover on semiconductors and conductors, because a hydrogen atom can migrate as a proton (H + ) and electron (e − ) pair. Protons can migrate over the support surface and electrons can transfer through the conduction band of material framework, which is thermodynamically feasible process [5] . In contrast to the cases of semiconductors and conductors, there have been ongoing debates on the existence of hydrogen spillover on insulating materials (SiO 2 , Al 2 O 3 and zeolite). It is noteworthy that most industrial catalysts are prepared by using these materials as a support because of their high thermochemical stability, regeneration feasibility, tunable acidity and low cost. Therefore, proving the existence and the catalytic functions of hydrogen spillover on these supports is very important in the catalysis field. Despite extensive studies on these metal oxides, the nature of spillover species, the migration mechanism, catalytic functions and even its existence remain topics of vigorous debate [5] . For a large part, this is a consequence of the lack of model catalysts that can provide direct evidences on the existence of hydrogen spillover and simplify the catalytic interpretation. In the conventional metal-supported catalysts, metal clusters are located on an open porous structure and hence organic reactants as well as H 2 can diffuse onto the metal surface in the course of the catalytic reaction. This allows the reactions to occur not only on the support surface (via hydrogen spillover) but also on the metal surface, thus leading to difficulty in decoupling the contributions from both pathways ( Fig. 1a ). Such ambiguity can be avoided by designing catalysts where metal clusters are selectively encapsulated in a dense support matrix so that only small H 2 can access but larger organic reactant cannot. Because organic molecules cannot diffuse to the encapsulated metal clusters, all catalytic activities can be directly attributed to the reaction between spillover hydrogen and organic molecules at the external surface of support matrix ( Fig. 1b ). Particularly, interesting examples are Pt in LTA zeolites (NaA and KA) that have very small pore apertures (0.3–0.4 nm) and hence selectively allow the diffusion of H 2 (0.29 nm) over various organic molecules [6] , [7] , [8] , [9] , [10] . Earlier catalytic studies using these materials, however, have not led to generally agreeable conclusion. Pt/NaA was reported to show negligible hydrogenation activities for isobutylene [6] and ethylbenzene [7] , indicating inappreciable catalytic function of hydrogen spillover. It was also reported that the isobutylene hydrogenation activity of Pt/KA is negligible but significantly increases when it is mixed with NaY and H-ZSM-5 (ref. 8) [8] . This was ascribed to hydrogen spillover from the Pt/KA to the NaY or H-ZSM-5 surface where the isobutylene was hydrogenated. Transmission electron micrographs (TEM) investigation showed, however, that some of the Pt particles were much larger than the zeolite cages and that part of the zeolite structure was damaged [5] , [8] . 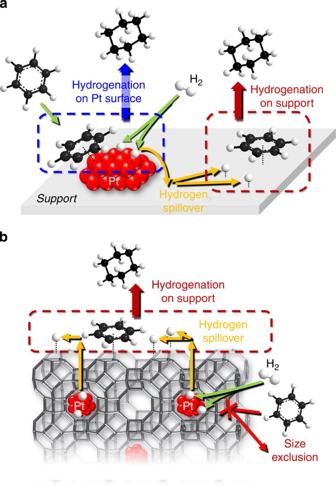Figure 1: Schematic representation for the hydrogenation pathways. (a) Conventional Pt catalysts supported on open porous supports and (b) Pt encapsulated in dense support matrix that allows selective diffusion of hydrogen over organic reactants. In the latter case, only hydrogenation on the support surface via hydrogen spillover is plausible. Figure 1: Schematic representation for the hydrogenation pathways. ( a ) Conventional Pt catalysts supported on open porous supports and ( b ) Pt encapsulated in dense support matrix that allows selective diffusion of hydrogen over organic reactants. In the latter case, only hydrogenation on the support surface via hydrogen spillover is plausible. Full size image The inconsistent interpretations in earlier reports can be explained in part by premature conclusions based on less rigorous characterizations, as well as by the possibility that important parameters governing the spillover phenomena may have been overlooked. It was pointed out that hydrogen spillover onto these non-reducible oxides such as SiO 2 , Al 2 O 3 and zeolite would be energetically improbable if there are no defect sites that can stabilize atomic hydrogen [5] . Defect sites generated from Brønsted acid sites (BAS, Si-OH-Al) [11] or other surface hydroxyls [12] , [13] , [14] , [15] , [16] may stabilize the atomic hydrogen, but their possible contributions have not been systematically investigated. Another important concern is the external surface area of the support matrix. Considering that the catalytic reaction via hydrogen spillover occurs only at the surface of the support matrix, the surface area would be highly important. In the case of Pt/LTA zeolite systems, LTA zeolite generally grows as a bulk crystallite (a few microns) and thus possesses extremely low external surface area (<5 m 2 g −1 ). Such low surface area would be insufficient to investigate or utilize hydrogen spillover even if the phenomenon indeed exists. In the present work, we synthesize Pt/NaA zeolite in the form of nanocrystals having varied surface areas while selectively encapsulating Pt clusters in the zeolite micropores. Because negatively charged aluminum sites in NaA zeolite are all charge-balanced by Na + ions, there are negligible amounts of -OH groups but we have mostly -O − Na + groups. To deliberately generate surface hydroxyls, the Pt/NaA materials are subsequently decationized in a controlled manner, which also results in the amorphization of zeolite framework. The catalytic investigations and density functional theory (DFT) calculations elucidate that surface hydroxyls, presumably BAS, play a crucial role for the surface migration of activated hydrogen. The catalysts working via hydrogen spillover show distinct chemoselectivity: they exhibit considerable activities for hydro-/dehydrogenation but virtually no hydrogenolysis activity compared with conventional Pt catalysts. This indicates that the catalysts can add or subtract H to or from organic molecules without breaking C-C bonds. Such distinct chemoselectivity may provide remarkable benefit in industrially important hydroconversions such as propane dehydrogenation to propylene, because an undesirable hydrogenolysis pathway producing light hydrocarbons of low value (for example, CH 4 and C 2 H 6 ) is greatly suppressed. Material synthesis and characterization Highly selective Pt encapsulation in NaA was attained by using a mercaptosilane-assisted metal encapsulation method [6] . To control the zeolite crystallite size of the Pt/NaA, varied amounts of polyethyleneglycol (PEG) were added into the zeolite synthesis gel as a crystal growth inhibitor [17] . The resultant samples were denoted as Pt/NaA- n , where n indicates the molar amount of PEG in the synthesis gel composition (see Methods). All the Pt/NaA- n samples were highly crystalline, showing the typical XRD pattern for a LTA structure ( Fig. 2a and Supplementary Fig. 1 ). The Brunauer-Emmett-Teller (BET) area of Pt/NaA- n samples analysed from N 2 adsorption at 77 K gradually increases with increasing n , which indicates that the addition of PEG can effectively decrease the zeolite crystallite size. Since N 2 diffusion into the NaA micropores is kinetically hindered at 77 K [18] , the BET area can be directly correlated to the external surface area of the zeolite crystallites. On the basis of unit cell information (cell dimension: 1.19 nm, Na 12 [Al 12 Si 12 O 48 ]) of NaA zeolite, we could estimate that the average crystallite size varies from 1,190 to 76 nm with the addition of PEG ( Table 1 ). TEM investigations ( Fig. 2d and Supplementary Fig. 2 ) revealed that Pt clusters in all the Pt/NaA- n samples are uniform in diameter (~1.0 nm). The Pt-Pt coordination number analysed from the extended X-ray absorption fine structure (EXAFS, Supplementary Table 1 ) for Pt/NaA-0 was 6.8±1.2, which corresponds to spherical Pt clusters having 1.0±0.4 nm diameter [19] . The cluster sizes determined by TEM and EXAFS are consistent with the diameter of a NaA α-cage (1.1 nm) [18] . H 2 and CO chemisorption at 323 K gave H/Pt and CO/Pt ratios between 0.52 and 0.67 for the Pt/NaA- n samples ( Table 1 ). If we assume the spherical morphology of Pt cluster, the Pt diameter (in nm) should be roughly the inverse of metal dispersion (that is, H/Pt or CO/Pt) [19] . It means that ~1.0 nm cluster should show H/Pt or CO/Pt values close to 1.0. The Pt/NaA- n samples showed the chemisorption values somewhat smaller than 1.0 (0.52< H/Pt or CO/Pt <0.67). This can be explained by the limited access of H 2 and CO to the Pt clusters tightly fitted in the small-pore zeolite structure [7] , [20] . 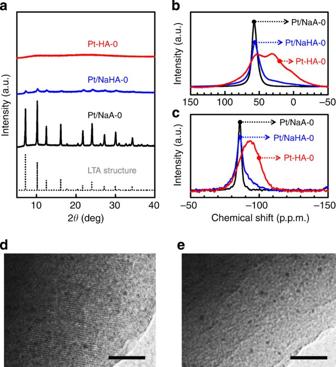Figure 2: Characterization of the Pt-encapsulated catalysts. (a) XRD patterns of Pt/ NaA-0 and decationized (amorphitized) samples (Pt/NaHA-0 and Pt/HA-0). (b)27Al and (c)29Si-NMR spectra for Pt/NaA-0, Pt/NaHA-0 and Pt/HA-0 samples. TEM images of (d) Pt/NaA-0 and (e) Pt/HA-0. Scale bars ind,eare 20 nm. The TEM images are representative of other TEM images (seeSupplementary Fig. 2) that showed similar and consistent features. Figure 2: Characterization of the Pt-encapsulated catalysts. ( a ) XRD patterns of Pt/ NaA-0 and decationized (amorphitized) samples (Pt/NaHA-0 and Pt/HA-0). ( b ) 27 Al and ( c ) 29 Si-NMR spectra for Pt/NaA-0, Pt/NaHA-0 and Pt/HA-0 samples. TEM images of ( d ) Pt/NaA-0 and ( e ) Pt/HA-0. Scale bars in d , e are 20 nm. The TEM images are representative of other TEM images (see Supplementary Fig. 2 ) that showed similar and consistent features. Full size image Table 1 Physicochemical properties of Pt catalysts. Full size table To investigate the effect of surface hydroxyls on hydrogen spillover, the Pt/NaA- n samples were ion-exchanged with controlled amounts of NH 4 + and calcined at 673 K. The resultant samples were denoted as Pt/NaHA- n and Pt/HA- n , depending on the degree of ion-exchange. The treatment resulted in decationization of Na + : the Na/Al ratio was decreased from 1.0 for Pt/NaA- n to 0.54–0.56 for Pt/NaHA- n and <0.10 for Pt/HA- n ( Table 1 ). The decationization led to a significant loss of zeolite crystallinity ( Fig. 2a ) because the NH 4 + form of highly aluminous LTA zeolite is unstable and collapsed (amorphitized) upon heat treatment [18] . The initial Pt/NaA- n samples showed single narrow peaks in both the 27 Al and 29 Si MAS NMR spectra ( Fig. 2b,c ), corresponding to tetrahedral Al [60 p.p.m.] and Si linked to four Al atoms (Si(4Al)) [−85 p.p.m. ], respectively. In clear contrast, the fully decationized Pt/HA- n showed three broad peaks ( Fig. 2b ) at 0, 25 and 60 p.p.m. in the 27 Al MAS NMR spectrum, which can be respectively assigned to octahedral, penta-coordinated and tetrahedral Al sites. The sample also showed a very broad peak centred at −95 p.p.m. in the 29 Si MAS NMR spectrum ( Fig. 2c ), which indicates heterogeneous formation of Si sites possessing lower numbers of surrounding Al atoms. The peak positions for Si with lower Al coordinations were previously assigned as Si(3Al) [−89 p.p.m. ], Si(2Al) [−95 p.p.m. ], Si(1Al) [−101 p.p.m. ], and Si(0Al) [−105 p.p.m.] [21] . The very broad peak centred at −95 p.p.m. (the same position for Si(2Al)) in the 29 Si MAS NMR spectrum indicates that roughly half of framework Al sites were dealuminated in Pt/HA- n compared with pristine Pt/NaA- n . The Pt/NaHA- n samples showed NMR spectra that are quite similar to those of pristine Pt/NaA- n . This indicates that minor fraction of Al (<20%) was dealuminated in Pt/NaHA- n . In the IR spectra, OH stretching band (3,000–3,800 cm −1 ) is almost invisible in Pt/NaA- n but becomes gradually pronounced as the degree of decationization increases ( Supplementary Fig. 3 ). The present results indicate that the decationization of Na + leads to amorphization of crystalline zeolite structure while generating surface hydroxyl groups. As shown by TEM images ( Fig. 2d,e , and Supplementary Fig. 2 ) and EXAFS analyses ( Supplementary Table 1 ), the size of encapsulated Pt clusters remained the same (~1.0 nm) upon the zeolite amorphization. The original cubic morphology of the NaA crystallites ( Supplementary Fig. 4 ) were retained (pseudomorphic transformation) and the BET surface areas decreased slightly (<20%, Table 1 ). These results indicate that zeolite amorphization does not change the mean Pt particle size but induces short-range atomic rearrangements of the zeolite into the amorphous aluminosilicate. The fully amorphitized Pt/HA- n samples showed negligible chemisorption of H 2 and CO (H/Pt and CO/Pt <0.02) at 323 K ( Table 1 ) despite that they still contain ~1.0 nm Pt clusters as confirmed by TEM and EXAFS. This reveals that Pt clusters are encapsulated in the amorphous aluminosilicate that is too dense to allow the diffusion of H 2 and CO (see the schematic model in Fig. 3 ). Surprisingly, the Pt/HA- n samples showed monotonically increasing H/Pt as the adsorption temperature was increased from 323 to 573 K ( Fig. 3c and Supplementary Fig. 5 ). Assuming ordinary exothermic adsorption processes, the adsorption capacity should monotonically decrease with increasing temperature, as observed for H 2 and CO chemisorption on the Pt/NaA- n and conventional Pt/SiO 2 catalyst ( Fig. 3a,d ). The adsorption behaviour of the Pt/HA- n samples is attributed to increased accessibility of H 2 onto the encapsulated Pt surface at elevated temperatures, since the penetration ability of H 2 molecules into the dense matrix can be increased because of the higher kinetic energy at elevated temperatures. In contrast, CO adsorption for the Pt/HA- n samples remained almost zero (<0.02) over the entire temperature range; this indicates that CO cannot diffuse in the amorphitized aluminosilicate matrix even at elevated temperatures because of its larger molecular size (0.38 nm) than H 2 (0.29 nm). The Pt/NaHA- n samples showed intermediate behaviour between the Pt/NaA- n and Pt/HA- n samples. The samples showed moderate H 2 chemisorption at 323 K, while they showed negligible CO chemisorption over the entire temperature range. The results reveal that amorphization transforms the zeolite into a less open aluminosilicate matrix imposing larger diffusional constraints, while a major portion of Pt clusters are still encapsulated as ~1.0 nm clusters. The increased diffusional constraints in the amorphitized samples were also confirmed by CO 2 (0.33 nm) adsorption at 273 K ( Supplementary Fig. 6 ). The Pt/NaA-0 showed 79 cm 3 g −1 (STP) CO 2 adsorption amount at 100 kPa. The adsorption amount significantly and gradually decreased as the degree of amorphization increased. In result, Pt/NaHA-0 showed 13 cm 3 g −1 and Pt/HA-0 showed 2 cm 3 g −1 adsorption amounts at the same pressure. The results again confirm that the amorphization transforms the NaA zeolite into a denser amorphous aluminosilicate. 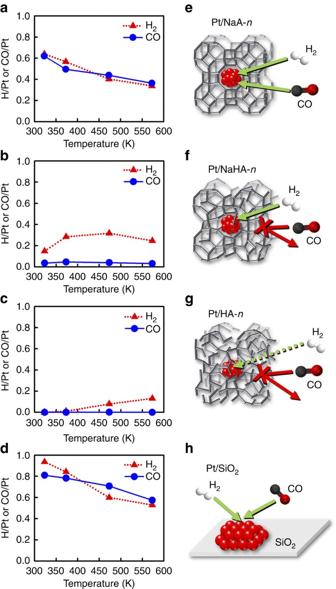Figure 3: H2and CO chemisorption at different adsorption temperatures. (a,e) Pt/NaA-0, (b,f) Pt/NaHA-0, (c,g) Pt/HA-0, and (d,h) Pt/SiO2. On the basis of the chemisorption data (a–d) and various analyses inFig. 2, the schematic catalyst structures were proposed (e–h). As the amorphization degree increases from Pt/NaA-nto Pt/HA-n, the zeolite is collapsed to a more amorphous and less open aluminosilicate structure imposing larger gas diffusional constraints. Figure 3: H 2 and CO chemisorption at different adsorption temperatures. ( a , e ) Pt/NaA-0, ( b , f ) Pt/NaHA-0, ( c , g ) Pt/HA-0, and ( d , h ) Pt/SiO 2 . On the basis of the chemisorption data ( a – d ) and various analyses in Fig. 2 , the schematic catalyst structures were proposed ( e – h ). As the amorphization degree increases from Pt/NaA- n to Pt/HA- n , the zeolite is collapsed to a more amorphous and less open aluminosilicate structure imposing larger gas diffusional constraints. Full size image Catalytic reactions Because all the Pt-encapsulated materials (totally nine samples: three different surface areas × three different hydroxyl concentrations) allow selective diffusion of H 2 over organic molecules, they can be used as a model catalyst for studying the catalytic functions of hydrogen spillover. To fully elucidate the catalytic functions of hydrogen spillover, we studied model reactions involving three different types of hydrogen transfer: (1) benzene hydrogenation to cyclohexane (H addition); (2) cyclohexane dehydrogenation to benzene (H subtraction); and (3) propane hydrogenolysis to methane and ethane (cleavage of C-C bond with H addition). The experimental details are given in Methods. The catalytic turnover rates (TOR, mol react mol Pt −1 s −1 ) were rigorously measured at a low conversion regime (<3%) to avoid heat transfer limitation. It should be noted that the catalytic turnover rate (TOR) in this work was calculated based on the total number of Pt rather than that of the accessible surface-Pt determined by H 2 or CO chemisorption at ambient temperature. This is because of the fully amorphitized Pt/HA- n samples showing almost zero H/Pt or CO/Pt values at ambient temperature ( Table 1 ), which leads to a scientifically meaningless TOR value of ‘infinity’ from the latter definition. Regardless of the surface area of aluminosilicates (or n ), the Pt/NaA- n samples exhibited negligible catalytic activities in benzene hydrogenation and cyclohexane dehydrogenation compared with Pt/SiO 2 ( Fig. 4a,b ). This indicates that Pt is selectively encapsulated in small zeolite micropores (aperture size: 0.40 nm), to which the organic reactants with larger kinetic diameters (benzene: 0.59 nm, cyclohexane: 0.60 nm) cannot access. The negligible catalytic activities also reveal that the catalytic contribution of hydrogen spillover is not visible in these materials. Our result is consistent with earlier reports showing that Pt/NaA is not active for the hydrogenation of organic molecules, and hence there is no indication of the catalytic contribution of hydrogen spillover [6] , [7] . In contrast, the amorphitized samples (Pt/NaHA- n and Pt/HA- n ) showed remarkably larger catalytic activities than the Pt/NaA- n samples in both hydrogenation and dehydrogenation ( Fig. 4a,b ). As proven from H 2 and CO chemisorption ( Fig. 3 ), Pt/NaHA- n and Pt/HA- n samples have less open aluminosilicate structures than Pt/NaA- n and impose more significant diffusion limitations for H 2 . It is worth remembering that the fully amorphitized Pt/HA- n samples allow H 2 diffusion only at elevated temperatures. Thus, the plausible explanation for the higher activities of amorphitized materials than Pt/NaA- n is facile migration of activated hydrogen (that is, hydrogen spillover) to the external surface of the aluminosilicate matrix. The results strongly indicate that the surface hydroxyls play a crucial role in the migration of activated hydrogen. The highest activities of Pt/NaHA- n among the three series of samples having different amorphization degrees are attributed to an optimal compromise between the diffusion rate of gaseous H 2 and the surface migration rate of activated hydrogen (the rate of hydrogen spillover) in the aluminosilicate matrix ( Fig. 4d ). 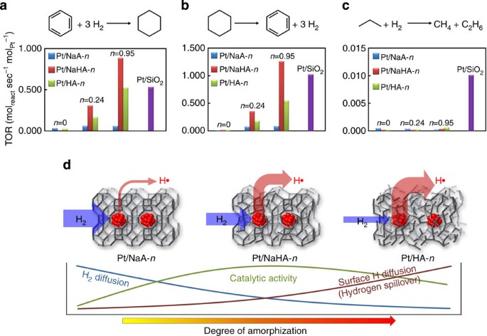Figure 4: Catalytic properties. Turnover rates (TOR) in (a) benzene hydrogenation (523 K, 473 kPa H2and 27 kPa benzene), (b) cyclohexane dehydrogenation (623 K, 94.3 kPa H2and 5.7 kPa cyclohexane) and (c) propane hydrogenolysis (643 K, 40 kPa H2, 10 kPa propane and 50 kPa He). It should be noted that all the TOR values in this work were calculated based on the total number of Pt rather than that of the surface-Pt determined by H2or CO chemisorption at ambient temperature. (d) A schematic representation of the diffusional and catalytic properties of Pt-encapsulated catalysts. Figure 4: Catalytic properties. Turnover rates (TOR) in ( a ) benzene hydrogenation (523 K, 473 kPa H 2 and 27 kPa benzene), ( b ) cyclohexane dehydrogenation (623 K, 94.3 kPa H 2 and 5.7 kPa cyclohexane) and ( c ) propane hydrogenolysis (643 K, 40 kPa H 2 , 10 kPa propane and 50 kPa He). It should be noted that all the TOR values in this work were calculated based on the total number of Pt rather than that of the surface-Pt determined by H 2 or CO chemisorption at ambient temperature. ( d ) A schematic representation of the diffusional and catalytic properties of Pt-encapsulated catalysts. Full size image The Pt-encapsulated samples showed enhanced benzene hydrogenation activities as the surface area of aluminosilicate matrix (or n ) increased ( Fig. 4a ). Dehydrogenation of cyclohexane ( Fig. 4b ) also showed the same trend. In the dehydrogenation, where hydrogen subtraction from organic molecules is involved instead of hydrogen addition, the catalytic activities are attributed to ‘reverse’ spillover, which corresponds to microscopic reversibility of hydrogen spillover phenomena [3] , [22] . In both reactions, the enhanced catalytic activities at larger surface area can be ascribed to an increased number of active sites on the support surface where spillover hydrogen can be added to or subtracted from the organic molecules. It is notable that the Pt/NaHA-0.95 sample with large surface area and an optimum amorphization degree showed the highest catalytic activities, even surpassing those of Pt/SiO 2 , which has a large accessible metal surface area (H/Pt=0.94, CO/Pt=0.81). This indicates that high catalytic activities in hydro-/dehydrogenation can be realized solely based on hydrogen spillover, if the nanostructure of the catalyst is properly designed. Notably even the amorphitized Pt/NaHA- n and Pt/HA- n samples having surface hydroxyls showed virtually switched-off activity for the hydrogenolysis of propane to methane and ethane ( Fig. 4c ). Pt/SiO 2 , having an open porous structure, showed markedly higher activity than these samples. A previous study using Pt/SiO 2 as a model catalyst showed a monotonic increase of TOR with decreasing Pt cluster size in a range of 1.7–7.1 nm (ref. 23 ). It was proposed that coordinatively unsaturated metal sites play an important role in the C-C bond breakage [23] , [24] . Because the Pt cluster sizes in the Pt-encapsulated catalysts and Pt/SiO 2 are comparable (~1.0 nm), as determined from the EXAFS analysis ( Supplementary Table 1 ), all the catalysts are expected to show similar hydrogenolysis activity if the reaction occurs on the Pt cluster surface. The present result indicates that the surface sites where the spillover hydrogen and propane react cannot break C-C bonds. The distinct chemoselectivity of Pt-encapsulated catalysts strongly supports that the catalysts operate via a non-conventional reaction mechanism (via hydrogen spillover). From a practical point of view, such selective hydro-/dehydrogenation function with suppressed hydrogenolysis activity would be highly beneficial in various industrial hydroconversions because hydrogenolysis produces light hydrocarbons of low value (for example, CH 4 and C 2 H 6 ). For instance, propane dehydrogenation is an important industrial route to produce propylene and it has become more important after the discovery of wet shale gas worldwide [25] . In this process, hydrogenolysis of propane is the main side reaction lowering the yield of propylene. We carried out propane dehydrogenation with Pt/NaHA-0.95 and Pt/SiO 2 catalysts (823 K, 80 kPa He, 10 kPa H 2 and 10 kPa propane). At the same propane conversion level of 26%, Pt/NaHA-0.95 showed 90% selectivity to propylene, which is markedly higher than that of Pt/SiO 2 (63%) due to the significantly suppressed hydrogenolysis activity. As a consequence of Pt encapsulation, the model catalysts also provide an additional advantage of extremely high thermal stability of Pt. For instance, the Pt clusters in Pt/NaA-0.95, Pt/NaHA-0.95 and Pt/HA-0.95 do not sinter even after harsh thermal treatment (H 2 atmosphere, 973 K for 12 h, Supplementary Fig. 7 ). In contrast, conventional Pt/SiO 2 showed significant sintering of Pt clusters (from 1.1 to 3.1 nm according to H 2 chemisorption). DFT calculations To provide insight into the long-range migration mechanism of the activated hydrogen, quantum mechanical (QM) DFT calculations were carried out. Although it has been roughly discussed that radical-type defect sites are likely to be involved during the spillover process onto non-reducible supports [5] , their equilibrium abundance is not believed to be sufficiently substantial to fully explain the observed catalytic activities. For example, the equilibrium concentration of defect sites such as ≡Si· or –Si(or Al)-O·would not be considerable even at high temperature due to the strong bond strength of Si-H or Si(or Al)O-H (~5 eV, Supplementary Table 2 ). In this regard, dynamic defect generation–annihilation paths are explicitly considered in the calculation of overall H migration mechanism to consider the equilibrium structure of aluminosilicate as being almost defect-free. We considered an aluminosilicate with an alternative arrangement of Si and Al (like pristine NaA zeolite) as our energetic reference state and used BAS possessing a substantial radical character [11] as the major mediator for hydrogen migration. This can be justified by the aforementioned NMR analyses indicating that the alternative linkage of Al and Si is mostly retained in Pt/NaHA- n ( Fig. 2b,c ). Even the fully amorphitized Pt/HA- n samples showed a sufficient presence (~50%) of framework Al. When the number of BAS in the aluminosilicates is sufficient to develop a percolated structure, a line path of BAS groups connecting the interior regime (where Pt is encapsulated) with the exterior regime (where organic molecules react) can be considered ( Fig. 5a ). In Fig. 5a , Al at the left-end is considered to be located at the external support surface and it is reasonably assumed to possess three covalent bonds with oxygen atoms. At this initial defect-free stage, a proton (H + ) in BAS can migrate in either of two different directions; over the Si atom (a barrier of 0.98 eV) or over the Al atom (1.97 eV). Considering the reaction temperature, only the former process seems plausible and would simultaneously produce two defect sites, [AlO 4 H 2 ] + and [AlO 4 ] − . The energy cost to generate this pair of defect sites is 0.49 eV. Once the defect pair of [AlO 4 H 2 ] + and [AlO 4 ] − is generated, the consecutive proton hopping over the Si atom can effectively migrate both [AlO 4 H 2 ] + and [AlO 4 ] − sites, where the QM migration barriers are only 0.70 eV for [AlO 4 H 2 ] + and 0.79 eV for [AlO 4 ] − ( Fig. 5b ). When cationic defect site finally migrates to the trivalent Al site at the external surface via the consecutive proton hopping, the Al possesses Lewis acidic character. DFT calculation showed that the Al site with Lewis acidic character can act as a binding site for unsaturated organic compounds due to the formation of a charge-transfer complex. 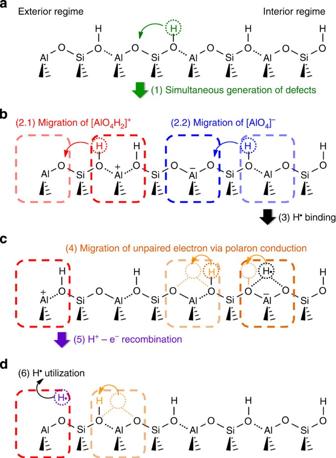Figure 5: Proposed mechanism for the hydrogen spillover. (a) Simultaneous generation of [AlO4H2]+and [AlO4]−defect sites by proton (H+) hopping. (b) Subsequent migration of [AlO4H2]+and [AlO4]−defect sites via consecutive H+hopping. (c) Addition of H radical (H·) to [AlO4]−defect site to form [AlO4]−H· via the formation of a three-centred bond (O-H-O), which can be regarded as Brønsted acid site distorted by the location of spatially localized unpaired electron (that is, polaron). (d) Migration of [AlO4]−H· site by transforming the adjacent O-H bond into the three-centred bond (O-H-O) (polaron conduction mechanism). When the unpaired electron eventually migrated to the cationic defect site, a proton recombines with the electron to generate H·. Additional detail is provided inSupplementary Figs 8–22. Figure 5: Proposed mechanism for the hydrogen spillover. ( a ) Simultaneous generation of [AlO 4 H 2 ] + and [AlO 4 ] − defect sites by proton (H + ) hopping. ( b ) Subsequent migration of [AlO 4 H 2 ] + and [AlO 4 ] − defect sites via consecutive H + hopping. ( c ) Addition of H radical (H·) to [AlO 4 ] − defect site to form [AlO 4 ] − H· via the formation of a three-centred bond (O-H-O), which can be regarded as Brønsted acid site distorted by the location of spatially localized unpaired electron (that is, polaron). ( d ) Migration of [AlO 4 ] − H· site by transforming the adjacent O-H bond into the three-centred bond (O-H-O) (polaron conduction mechanism). When the unpaired electron eventually migrated to the cationic defect site, a proton recombines with the electron to generate H·. Additional detail is provided in Supplementary Figs 8–22 . Full size image Our QM calculation shows that the binding of the H radical (H·) at the bridge-site of two oxygen atoms of [AlO 4 ] − is favourable by 0.09 eV via the formation of a three-centred bond (O-H-O). This indicates that the [AlO 4 ] − site can serve as a good H· accepting site, yielding [AlO 4 ] − H· ( Fig. 5c ). We can regard the formation of three-centred bond ([AlO 4 ] − H·) as a local structural distortion from the original BAS site [AlO 4 ] − H + due to the location of spatially localized unpaired electron, that is, polaron. Then, the unpaired electron localized at [AlO 4 ] − H· can easily migrate into the nearest BAS site by changing the conventional O-H bond into the three-centred O-H-O bond (deforming the nearest BAS site), which is often referred as a polaron conduction mechanism. The barrier for this polaron conduction process is estimated as 0.60–0.69 eV ( Supplementary Fig. 8 ). When the unpaired electron eventually migrates into the cationic defect site via a number of migrations, the proton recombines with the electron, yielding H· that can be easily transferred to organic molecules adsorbed at the external Al sites for hydrogenation reaction ( Fig. 5d ). Summing up, the proposed reaction mechanism migrates the activated hydrogen via a proton relaying (similar to Grotthuss mechanism), while an electron migrates on the zeolite surface via exchanging local bond connectivities (O-H and O-H-O bond) to induce polaron-type conduction; therefore, the hydrogen spillover onto the non-reducible aluminosilicate becomes energetically viable (overall activation energy <0.98 eV, Supplementary Fig. 9 ) without involving a series of homolytic bond dissociation and formation processes (>~5 eV). Although our DFT calculations considered BAS (Si-OH-Al) as a main mediator for the migration of H atom, any type of proton source that can relay the proton hopping such as silanols (-Si-OH) is able to participate in the proposed mechanism. All of the present intriguing observations cannot be rationally explained by any other factors than hydrogen spillover. It may be argued that minor amounts of non-encapsulated external Pt species (too minor to be detected by chemisorption, EXAFS and TEM) can account for the catalytic results. However, it should be emphasized again that the catalytic turnover rates in this work were calculated based on the total number of Pt rather than that of Pt accessible by H 2 or CO. For the minor external Pt species to cover the entire catalytic activities observed in the hydro-/dehydrogenation reactions, their specific activity should be orders of magnitude higher than ordinary Pt species. Considering that the specific activities of Pt in hydro-/dehydrogenation have been reported to be relatively insensitive to Pt cluster size and shapes [24] , the assumption of the existence of ‘super-active’ Pt is unreasonable. Furthermore, the distinct chemoselectivity (suppressed hydrogenolysis) and the remarkable dependence of catalytic activity on the hydroxyl concentration of support surface cannot be explained by the conventional reaction mechanism on metal surface. We expect that the present observations can be used to design advanced hydroprocessing catalysts with enhanced catalytic activities, tolerance against thermal sintering and distinct chemoselectivity. Material synthesis Pt-encapsulated NaA zeolites were prepared by crystallization of the Pt-containing aluminosilicate gel in the presence of (3-mercaptopropyl)trimethoxysilane at 353 K 6 . In a typical synthesis, 0.8 g (3-mercaptopropyl)trimethoxysilane and 2.3 g NaOH were dissolved in 8 g deionized H 2 O. A solution of 0.5 g H 2 PtCl 6 in 4.6 g H 2 O was added dropwise into the previous solution while stirring vigorously. Eighteen grams colloidal silica (Ludox-AS30, 30 wt% SiO 2 ) was then added and the mixture was heated to 353 K under stirring until clear Na-silicate solution was obtained. Varied amounts of PEG (Sigma-Aldrich, avg M n ; 1,450) were added to the silicate solution and stirred at 353 K for 1 h. Finally, 11.5 g NaAlO 2 dissolved in 16 g H 2 O was added to the aforementioned solution. The final synthesis gel composition was 1.5 SiO 2 : 1.0 Al 2 O 3 : 1.8 Na 2 O: 38 H 2 O: 0.016 H 2 PtCl 6 : 0.064 (3-mercaptopropyl)trimethoxysilane: n PEG, where n was varied from 0 to 0.95. The synthesis gels were hydrothermally crystallized at 353 K for 48 h, filtered and thoroughly washed with deionized water until the pH of the filtrated solution becomes 8. The samples were dried at 373 K for 24 h. The as-synthesized samples were sequentially treated in dry air and H 2 at 673 K (flow rate 200 ml min −1 g −1 ) for 2 h to remove organic species and to form reduced Pt clusters in the zeolite micropores.The resultant samples were denoted as Pt/NaA- n , where n indicates the molar amount of PEG in the synthesis gel composition. The Pt/NaA- n samples were decationized by the ion-exchange with NH 4 + and subsequent air calcination at 673 K for 2 h. For the synthesis of partially decationized Pt/NaHA- n samples, 1 g of Pt/NaA- n samples was ion-exchanged with the 14 ml of 0.5 M NH 4 NO 3 solution for 6 h at room temperature. For the synthesis of fully decationized Pt/HA- n samples, 1 g of Pt/NaA- n sample was ion-exchanged three times with the 140 ml of 0.5 M NH 4 NO 3 solution. Pt/SiO 2 sample was prepared via conventional incipient wetness impregnation of the aqueous solution of Pt(NH 3 ) 4 (NO 3 ) 2 (Sigma-Aldrich) into the mesoporous silica gel (Davisil Grade 636, Sigma-Aldrich). The impregnated sample was dried at 373 K for 24 h, calcined in dry air at 523 K for 2 h (200 ml min −1 g −1 ) and reduced in H 2 at 673 K for 2 h (200 ml min −1 g −1 ). Characterization Elemental analyses were carried out by using inductively coupled plasma atomic emission spectroscopy (ICP-AES) using iCAP-6500 (Thermo elemental). Powder X-ray diffraction (XRD) patterns were recorded using a D2-phaser (Bruker) equipped with Cu radiation (30 kV, 10 mA) and LYNXEYE detector. N 2 adsorption/desorption isotherms were measured using a BEL-Sorp-max (BEL Japan) volumetric analyzer at the liquid N 2 temperature (77 K). Before the adsorption measurement, all the samples were degassed at 623 K for 6 h, and the specific surface areas were determined in a P/P 0 range between 0.05 and 0.20, using BET equation. Scanning electron micrographs were taken with a Magellan400 (FEI) at a low landing energy (1 kV) without crushing or metal coating. TEM were collected by JEM-2100F (JEOL) at 200 kV acceleration voltages after mounting the samples on a copper grid (300 square mesh) using ethanol dispersion. Solid-state NMR spectra were recorded on a Bruker Avance 400 spectrometer equipped with a widebore 9.4T magnet, operating at a Larmor frequency, υ 0 , of 104.3 MHz for 27 Al and 79.5 MHz for 29 Si. Samples were packed inside 4 and 7 mm rotors, and MAS rates were 15 kHz and 5 kHz, respectively. 27 Al MAS NMR spectra were recorded with rf-field strengths of 50 kHz, recycle delay of 1 s and 90° solid pulse of 5 μs. 29 Si MAS NMR spectra were recorded with high power 1 H decoupling, rf-field strengths of 23.8 kHz, recycle delay of 25 s and 90° solid pulse of 7.6 μs. Chemical shifts were reported in p.p.m. relative to an external standard of 1 M aqueous Al(NO 3 ) 3 solution for 27 Al and 4,4-dimethyl-4-silapentane-1-sulphonic acid for 29 Si. H 2 and CO chemisorption isotherms were measured with ASAP2020 (Micromeritics) adsorption volumetric analyzer. H 2 (99.999%) and CO (99.9%) gases were used as received. Before adsorption measurement, all the samples were re-reduced at 673 K flowing H 2 (200 ml min −1 g −1 ) for 3 h, followed by evacuation for 3 h at the same temperature. Adsorption measurements were carried out at 323, 373, 473 and 573 K in the pressure range of 0.3–60 kPa. The chemisorption amounts were determined by extrapolation of the high-pressure linear portion (10–30 kPa) of the isotherm to zero pressure. CO 2 adsorption isotherms were measured using ASAP2050 (Micromeritics) adsorption volumetric analyzer at 273 K. Before the adsorption measurement, all the samples were degassed at 623 K for 6 h and the gas adsorption quantities were measured upto atmospheric pressure (~100 kPa). X-ray absorption spectra of Pt L 3 edge were measured in a transmission mode at Pohang Accelerator Laboratory (7D-XAFS beamline). Before the experiments, c.a. 0.3 g of sample was pressurized into the self-standing pellets (13 mm diameter) and re-reduced at 673 K in the in situ XAFS cells equipped with aluminum window of 0.05 mm thickness. EXAFS data were analyzed using ATHENA and ARTEMIS programs, interfaces for the IFEFFIT and FEFF codes. After background removal, the absorption spectra were Fourier-transformed over a k range of 3.6–13.7 Å −1 . Average coordination numbers of Pt clusters were obtained from EXAFS fits using ARTEMIS, and the size of the Pt clusters were determined from calculated average coordination numbers for spherical fcc Pt clusters of varying sizes [19] . For FT-IR measurement, Pt/NaA-0.95, Pt/NaHA-0.95 and Pt/HA-0.95 samples were pressed into a self-supporting wafer (11 mg cm −2 ). Before the IR measurements, each sample was degassed at 673 K for 4 h in a vacuum and cooled to room temperatrue in an in situ IR cell. After cooling to room temperature, IR spectra were collected using an FT-IR spectrometer (Thermo Nicolet NEXUS 470) with 128 scans and 4 cm −1 resolution in the 4,000–2,000 cm −1 range. Catalytic measurements All the reactions were carried out in a stainless steel (10.9 mm diameter) continuous down-flow fixed-bed reactor connected to an online gas chromatography. The catalysts were pressed into pellets without any diluents at 400 bar, crushed, sieved (75–100 mesh) and then physically mixed with quartz particles (75–100 mesh) before the catalytic measurements. The catalysts were pretreated at 673 K under flowing H 2 before the catalytic reactions. In all reactions, the catalytic turnover rates (TOR, mol react mol Pt −1 s −1 ) were measured at low conversion regime (<3%) to avoid heat transfer limitation. The reaction conditions are as follows: benzene hydrogenation (523 K, 473 kPa H 2 , and 27 kPa benzene); cyclohexane dehydrogenation (623 K, 94.3 kPa H 2 , and 5.7 kPa cyclohexane); propane hydrogenolysis (643 K, 50 kPa He, 40 kPa H 2 and 10 kPa propane). Propane dehydrogenation to propylene (823 K, 80 kPa He, 10 kPa H 2 and 10 kPa propane) was carried out with Pt/NaHA-0.95 and Pt/SiO 2 catalysts. The product selectivity was compared at the same propane conversion level of 26% by controlling the space velocity (0.33 and 0.27 mol react mol Pt −1 s −1 for Pt/NaHA-0.95 and Pt/SiO 2 , respectively). Computational methods Quantum mechanic (QM) calculations were carried out using the M06-2X flavour of hybrid DFT [26] combined with LACVP** basis set [27] by using Jaguar 7.6 program [28] . To mimic the infinitely long-chain of BAS at the zeolite surface, a ring-shaped structure composed of 8T (Si and Al) atoms is taken from the pore aperture of NaA system (ICSD 9326) ( Supplementary Fig. 10 ). This model structure consists of alternative arrangements of Al and Si atoms bridged through either an oxygen atom or an OH group (that is, BAS), and each Al or Si atom is coordinated by four oxygen atoms. The oxygen atoms located outside the ring are hydrogen terminated, leading to the chemical composition of Al 4 H 20 Si 4 O 24 . On the basis of this idealized and defect-free model structure, the energetics at each reaction step were calculated by optimizing the geometry under the constraint fixing the location of outer eight oxygen atoms as in the zeolite crystal structure. This enables us to include the ring strain of rigid zeolite structure during our energetic calculations. Transition state is optimized by following the eigenvector of the Hessian matrix with the largest negative eigenvalue, and it is confirmed by calculating the presence of one additional imaginary vibrational frequency except for the other imaginary frequencies originated from the constraint in positions of the outer oxygen atoms. Mulliken spin analysis [29] is employed to identify whether the character of H atom is protonic or radical-like. How to cite this article: Im, J. et al. Maximizing the catalytic function of hydrogen spillover in platinum-encapsulated aluminosilicates with controlled nanostructures. Nat. Commun. 5:3370 doi: 10.1038/ncomms4370 (2014).